Anisotropic magnetoresistance in an antiferromagnetic semiconductor Recent studies in devices comprising metal antiferromagnets have demonstrated the feasibility of a novel spintronic concept in which spin-dependent phenomena are governed by an antiferromagnet instead of a ferromagnet. Here we report experimental observation of the anisotropic magnetoresistance in an antiferromagnetic semiconductor Sr 2 IrO 4 . Based on ab initio calculations, we associate the origin of the phenomenon with large anisotropies in the relativistic electronic structure. The antiferromagnet film is exchange coupled to a ferromagnet, which allows us to reorient the antiferromagnet spin-axis in applied magnetic fields via the exchange spring effect. We demonstrate that the semiconducting nature of our AFM electrode allows us to perform anisotropic magnetoresistance measurements in the current-perpendicular-to-plane geometry without introducing a tunnel barrier into the stack. Temperature-dependent measurements of the resistance and anisotropic magnetoresistance highlight the large, entangled tunabilities of the ordinary charge and spin-dependent transport in a spintronic device utilizing the antiferromagnet semiconductor. A tunnelling anisotropic magnetoresistance (TAMR) has been previously reported in devices with an antiferromagnetic (AFM) metal electrode on one side and a non-magnetic metal on the other side of a tunnel barrier [1] , [2] , [3] , [4] , [5] . A room-temperature memory device has been realized utilizing the anisotropic magnetoresistance (AMR) of an AFM metal resistor for the electrical read-out of the AFM memory state [6] . These results have experimentally confirmed the viability of the proposal for utilizing spin-orbit coupled AFM metals in spintronic devices [7] . There are, however, fundamental physical limitations for metallic magnets, which may make them impractical to realize the full potential of spintronics. In particular, metals are unsuitable for transistor and information processing applications or for photonics. The synthesis of semiconductors with high-temperature ferromagnet (FM) ordering of spins, which would simultaneously enable the conventional tunability of electronic properties and spintronic functionalities, remains a significant challenge [8] . On the other hand, robust AFM ordering occurs much more frequently in nature than FM ordering, particularly in conjunction with semiconducting electronic structure [9] , [10] . Recent studies have identified several candidate AFM semiconductor materials, ranging from AFM counterparts of common zinc-blende or half-Heusler compound semiconductors [11] , [12] , [13] , [14] to perovskite semiconductor-AFM oxides [15] , [16] , [17] , [18] , [19] . A particular focus in this materials research has been on the preparation of thin epitaxial films and heterostructures [11] , [13] , [18] , [19] as a prerequisite for the envisaged spintronic devices. In the following, we make the step from the materials science to spintronics by observing the semiconductor-AFM AMR phenomenon in a heterostructure comprising Sr 2 IrO 4 (SIO). A Mott gap opens in SIO as a consequence of electron correlations, AFM order and strong spin-orbit coupling introduced by Ir [15] , [16] , [17] . The strong spin-orbit coupling makes SIO a favourable semiconductor AFM for observing the relativistic anisotropic magnetotransport phenomena, reminiscent of the TAMR experiments in the metal AFM IrMn [1] , [3] , [4] , [5] . We recall that the key signature of these relativistic anisotropic phenomena is that they are an even function of the microscopic magnetic moment vector, which makes them equally present in spin-orbit-coupled AFMs as in FMs. 7 Our observation of the AMR in an AFM semiconductor opens a new path for integrating semiconducting and spintronic phenomena and functionalities. Experimental observation of the AMR in the AFM semiconductor We have previously demonstrated the synthesis of high-quality epilayers of the semiconductor-AFM SIO on SrTiO 3 (STO) substrates using pulsed laser deposition [18] and demonstrated that the SIO films have semiconductor transport characteristics [18] , [19] . To allow for the rotation of the AFM spin-axis via the FM-AFM exchange spring effect [20] , we have prepared for the present study a heterostructure comprising an epitaxial 12 nm thick film of a FM metal La 2/3 Sr 1/3 MnO 3 (LSMO) inserted between a (001)STO single-crystalline substrate and a 6-nm thick film of the AFM semiconductor SIO. The high epitaxial quality of our LSMO/SIO heterostructure is illustrated in the scanning transmission electron microscopy is included in the detailed discussion of the structural quality and magnetic characteristics of our epilayers, which is presented in the Supplementary Figs 1–3 and Supplementary Notes 1–3 . Here we summarize that atomic force microscopy of the top SIO surface indicates that the multilayer preserved the substrate root-mean-square roughness below one unit cell. Both LSMO and SIO grow c axis oriented ([001]STO//[001]LSMO//[001]SIO) with an in-plane epitaxial relationship [100]STO//[100]LSMO//[110]SIO. The detected splitting of the zero-field-cooled and field-cooled magnetization curves below T* ~100 K is consistent with the canted AFM ground state of SIO [15] . The Néel temperature T N ~ T * is smaller than the bulk value (240 K), which is expected for a 6-nm thin SIO film. In Fig. 1a we compare the temperature-dependent transport characteristics of our LSMO/SIO device measured in the current-perpendicular-to-plane (CPP) and in the current-in-plane (CIP) geometries (see Supplementary Figs 4 and 5 and Supplementary Notes 4 and 5 for further details on transport measurements). In the CPP geometry, the electrical current I is driven from a contact patterned on top of the SIO epilayer vertically through the 6-nm width of the SIO film and then laterally along the [100] crystal axis over a macroscopic distance of 2.5 mm. In the CIP geometry, the current flows only in the plane of the epilayers between lateral contacts separated by 5 mm. The temperature dependence of the resistivity is vastly different in the two configurations. The CIP geometry is governed by the conduction through the metal LSMO over the entire temperature range. On the other hand, the CPP measurement confirms semiconducting transport through the SIO film as previously seen in experiments in bare epilayers of SIO [18] . At low temperatures, the vertical transport path through the semiconducting SIO film dominates the total resistance of the LSMO/SIO stack in the CPP geometry. 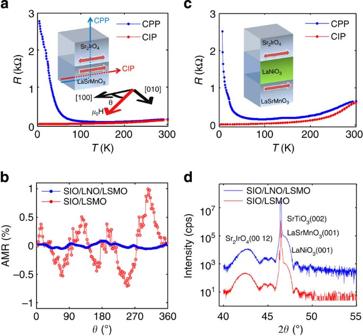Figure 1: Anisotropic magnetoresistance (AMR) in the antiferromagnetic Sr2IrO4(SIO) semiconductor. (a) Resistance as a function of temperature measured in the La2/3Sr1/3MnO3(LSMO)/SIO sample in the current-perpendicular-to-plane (CPP) and in the current-in-plane (CIP) geometries showing the semiconducting SIO and metal LSMO, respectively. Inset shows a sketch of the stack and transport measurement geometries. (b) Resistance measurement in an in-plane rotating magnetic field of 100 mT in the LSMO/SIO stack compared with the LSMO/LaNiO3(LNO)/SIO control. The SIO AMR is observed in the LSMO/SIO sample but not in the control LSMO/LNO/SIO sample at 100 mT or at higher applied fields. (c) CPP and CIP electrical resistance measured in the control LSMO/LNO/SIO sample indicating that LSMO is metallic and that the SIO layer has comparable electrical resistance and the same semiconducting character as in the LSMO/SIO stack. Inset shows a sketch of the control sample in which a 10-unit cell (4 nm) paramagnetic metal LNO is inserted between the LSMO and SIO layers in order to break the FM-AFM coupling. (d) X-ray diffraction patterns of the LSMO/SIO and LSMO/LNO/SIO samples confirming the presence of the SIO in the control LSMO/LNO/SIO stack with the same layer thickness and crystal quality as in the LSMO/SIO sample. Figure 1: Anisotropic magnetoresistance (AMR) in the antiferromagnetic Sr 2 IrO 4 (SIO) semiconductor. ( a ) Resistance as a function of temperature measured in the La 2/3 Sr 1/3 MnO 3 (LSMO)/SIO sample in the current-perpendicular-to-plane (CPP) and in the current-in-plane (CIP) geometries showing the semiconducting SIO and metal LSMO, respectively. Inset shows a sketch of the stack and transport measurement geometries. ( b ) Resistance measurement in an in-plane rotating magnetic field of 100 mT in the LSMO/SIO stack compared with the LSMO/LaNiO 3 (LNO)/SIO control. The SIO AMR is observed in the LSMO/SIO sample but not in the control LSMO/LNO/SIO sample at 100 mT or at higher applied fields. ( c ) CPP and CIP electrical resistance measured in the control LSMO/LNO/SIO sample indicating that LSMO is metallic and that the SIO layer has comparable electrical resistance and the same semiconducting character as in the LSMO/SIO stack. Inset shows a sketch of the control sample in which a 10-unit cell (4 nm) paramagnetic metal LNO is inserted between the LSMO and SIO layers in order to break the FM-AFM coupling. ( d ) X-ray diffraction patterns of the LSMO/SIO and LSMO/LNO/SIO samples confirming the presence of the SIO in the control LSMO/LNO/SIO stack with the same layer thickness and crystal quality as in the LSMO/SIO sample. Full size image The central result of our work is shown in Fig. 1b . At sufficiently low temperatures (4.2 K in Fig. 1b ), we apply an external in-plane magnetic field of an amplitude 100 mT and observe an AMR=[ R ( θ )− R (0)]/ R (0) signal in the CPP geometry while varying the field angle θ measured from the [100] axis, as defined in Fig. 1a . The field is much smaller than typical exchange fields in AFM oxides with super-exchange induced magnetic order and much larger than the coercive field of LSMO, which is approximately 5 mT at 4.2 K. The FM moments in LSMO follow the applied magnetic field angle and drag the AFM moments in SIO via the exchange spring effect at the FM/AFM interface. The resulting reorientation of the SIO AFM spin-axis produces the semiconductor-AFM AMR signal observed in Fig. 1b . We point out that we designed our stack with the small thickness of SIO to maximize the exchange-spring effect of the FM on the AFM [21] and to maximize the uniformity of the reorientation of the AFM spin-axis through the SIO epilayer. To confirm that the AMR signal in Fig. 1b does not originate from the transport through LSMO and that magnetic field does not couple directly to the AFM moments in SIO, we present in Fig. 1b–d control experiments in an epitaxial stack in which a non-magnetic LaNiO 3 (LNO) metal film of thickness 4 nm is inserted between the SIO and LSMO. Similar to the LSMO/SIO stack, a metallic temperature-dependent resistivity is observed in the LSMO/LNO/SIO sample in the CIP geometry and semiconducting transport characteristics in the CPP geometry (compare Fig. 1a,c ). The two samples have also comparable crystal quality as shown in Fig. 1d and magnetic characteristics (see Supplementary Fig. 6 and Supplementary Note 6 ). The difference between the two heterostructures is that LNO breaks the FM-AFM interlayer exchange coupling. As a result, the low-temperature ~1% CPP AMR signal seen in the LSMO/SIO sample is diminished in the control SIO/LNO/LSMO stack with uncoupled AFM and FM layers ( Fig. 1b ). This implies that transport though LSMO with rotating FM moments in the applied rotating magnetic field is not producing the AMR signal seen in Fig. 1b for the LSMO/SIO sample. Moreover, the measurements in the control LSMO/LNO/SIO sample confirm that any direct effect of the applied rotating magnetic field on the SIO magnetoresistance in our experiments is negligible compared with the AMR because of the AFM spin-axis reorientation via the LSMO/SIO exchange spring (For further discussion on the absence of a direct coupling of the applied magnetic field to the AFM moments in our SIO films, see Supplementary Information . ). Temperature dependence of the AMR signals In Fig. 2a–c and e–g we compare field-angle-dependent AMR data at μ 0 H =100 mT as a function of temperature detected in the CPP and CIP measurement configurations. In both cases, the current–voltage ( I-V ) characteristics remain Ohmic in the entire temperature range from room temperature to 4.2 K, as illustrated by the 4.2 K I-V data shown in Fig. 2d,h and d I/ d V data shown in Supplementary Fig. 7 and Supplementary Note 7 . At high temperature and for the CIP transport geometry ( Fig. 2e ), we observe the typical AMR of a FM material [22] . In a rotating in-plane magnetic field of strength larger than the coercive field, the FM moment m in LSMO follows μ 0 H . In the CIP transport geometry, this implies that the in-plane angle θ between m and the electrical current I// [100] vary, which results in the observed AMR signal proportional to sin(2 θ ). The observation that the resistance for I // m is smaller than for I ⊥ m in LSMO is in agreement with the previous report on the AMR in a similar FM manganite material La 2/3 Ca 1/3 MnO 3 (ref. 23 ). As LSMO is a FM metal with high ordering temperature, in the explored temperature range of Fig. 2e–g , the CIP AMR of LSMO is weakly temperature dependent. The observed small departure from the smooth sin(2 θ ) angular dependence at low temperatures is caused by an enhanced coercivity of LSMO when decreasing temperature (see corresponding magnetization data in Supplementary Fig. 6 ). 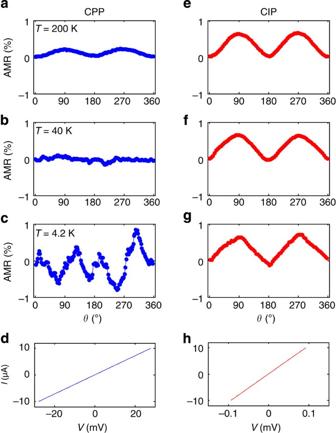Figure 2: Comparison of the temperature-dependent anisotropic magnetoresistance (AMR) signals of Sr2IrO4(SIO) and La2/3Sr1/3MnO3(LSMO) andI-Vcharacteristics of the heterostructure. AMR as a function of the temperature for the current-perpendicular-to-plane (CPP) and current-in-plane (CIP) transport geometries in a 100-mT in-plane rotating magnetic field. (a–c) In the CPP geometry, we observe three distinct temperature regimes of the device operation: at high temperatures, the AMR is dominated by the metal FM LSMO; at intermediate temperatures, no AMR is observed and at sufficiently low temperatures, the observed AMR signal is due to the antiferromagnetic semiconductor SIO. (e–g) In the CIP measurements, the LSMO AMR is probed. At higher temperatures, the sin(2θ) AMR is observed, at intermediate temperatures, belowTN, the coupling to SIO produces a small departure from the sin(2θ) dependence due to the enhanced LSMO coercivity. (d,h) OhmicI-Vcharacteristics measured at 4.2 K in the CPP and CIP geometries, respectively. Figure 2: Comparison of the temperature-dependent anisotropic magnetoresistance (AMR) signals of Sr 2 IrO 4 (SIO) and La 2/3 Sr 1/3 MnO 3 (LSMO) and I - V characteristics of the heterostructure. AMR as a function of the temperature for the current-perpendicular-to-plane (CPP) and current-in-plane (CIP) transport geometries in a 100-mT in-plane rotating magnetic field. ( a – c ) In the CPP geometry, we observe three distinct temperature regimes of the device operation: at high temperatures, the AMR is dominated by the metal FM LSMO; at intermediate temperatures, no AMR is observed and at sufficiently low temperatures, the observed AMR signal is due to the antiferromagnetic semiconductor SIO. ( e – g ) In the CIP measurements, the LSMO AMR is probed. At higher temperatures, the sin(2θ) AMR is observed, at intermediate temperatures, below T N , the coupling to SIO produces a small departure from the sin(2θ) dependence due to the enhanced LSMO coercivity. ( d , h ) Ohmic I-V characteristics measured at 4.2 K in the CPP and CIP geometries, respectively. Full size image AMR measurements in the CPP geometry are shown in Fig. 2a–c . At 200 K, we observe AMR~sin(2 θ ) ascribed to the LSMO as in Fig. 2e . The amplitude of the AMR is suppressed in the CPP geometry because of a comparable contribution to the measured resistance from a signal arising from the vertical transport path through the SIO film, which is non-magnetic at 200 K (see Supplementary Fig. 6 and Supplementary Note 6 ). At 40 K ( Fig. 2b ), the resistance of the short vertical path through the semiconducting SIO becomes dominant (see Supplementary Fig. 7 and Supplementary Note 7 ) and the AMR is diminished. Remarkably, when sufficiently below the Néel temperature of SIO (see Fig. 2c with 4.2 K data), the AMR signal increases again. As the resistance in the CPP geometry at these low temperatures is completely dominated by the vertical transport path through the SIO film, the observed AMR signal originates from the semiconductor-AFM layer. Detailed comparison of the AMR in the SIO and LSMO A clear signature of the distinct origin of the low-temperature AMR is the higher harmonic component of the SIO AMR signal as compared with the ~sin(2 θ ) AMR of the metal-FM LSMO. To highlight this point, we compare in Fig. 3a,b polar plots of the CPP AMR owing to SIO and CIP AMR owing to LSMO at 4.2 K and 350 mT. In Fig. 3c,d we show complete resistance maps, which were all collected after field-cooling the sample from 300 to 4.2 K in a 350 mT magnetic field applied along the in-plane angle θ =90°. With the temperature maintained at 4.2 K, subsequent field-rotation AMR measurements were performed at magnetic fields of strength varying from 350 to 5 mT. The polar plots in Fig. 3 and the resistance maps in Fig. 3c,d confirm the distinct phenomenology of the CPP AMR owing to SIO and the CIP AMR owing to LSMO. 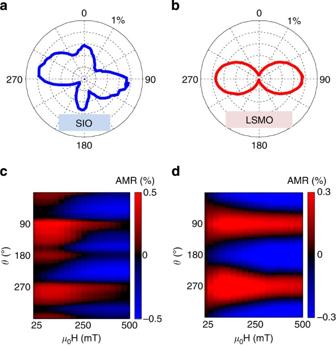Figure 3: Comparison of the anisotropic magnetoresistance (AMR) in Sr2IrO4(SIO) and La2/3Sr1/3MnO3(LSMO). (a,b) Polar plots corresponding to AMR experiments in a 350-mT in-plane rotating field and temperature 4.2 K. The LSMO AMR shows the sin(2θ) behaviour at this large magnetic field. The SIO AMR has a distinct, higher harmonic component. (c,d) Field-rotation AMR maps demonstrating the coupling of the LSMO and SIO moments. Figure 3: Comparison of the anisotropic magnetoresistance (AMR) in Sr 2 IrO 4 (SIO) and La 2/3 Sr 1/3 MnO 3 (LSMO). ( a , b ) Polar plots corresponding to AMR experiments in a 350-mT in-plane rotating field and temperature 4.2 K. The LSMO AMR shows the sin(2θ) behaviour at this large magnetic field. The SIO AMR has a distinct, higher harmonic component. ( c , d ) Field-rotation AMR maps demonstrating the coupling of the LSMO and SIO moments. Full size image The presence of the exchange-coupling between LSMO and SIO in the LSMO/SIO stack is apparent form the strong increase of the coercivity of LSMO at T < T N . This marked broadening of the hysteresis loop is absent in bare LSMO films or in the LSMO/LNO/SIO control structure (see Supplementary Fig. 6 ). The strong enhancement of the coercivity of LSMO in the LSMO/SIO stack, therefore, provides another evidence for the exchange-spring-induced rotation of the AFM spin-axis in our AMR measurements in SIO. We also note that the hysteresis loop measured at 4 K in the LSMO/SIO sample shows a small but clearly visible exchange-bias shift. This provides an additional confirmation of the presence of the exchange coupling at the LSMO/SIO interface. In Fig. 4a,b we compare the magnetoresistance, ΔR ( μ 0 H )/ R (0), at 4.2 K for the CPP and CIP transport measurements. The experiments were performed after field-cooling the sample in a magnetic field applied at the angle θ =90° and subsequently sweeping the field along θ =90° (red curves) or θ =180° (black curves). In the CIP and CPP transport geometries, the ΔR ( μ 0 H )/ R (0) data display closely related features, confirming that the SIO layer response follows the magnetization of LSMO. The coupling between the AFM and FM layers is particularly evident in the θ =180° field-sweep data. Here the CIP transport measurement shows a pronounced hysteretic double peak that signals an abrupt magnetic domain reconfiguration in LSMO. The observation that ΔR ( μ 0 H )/ R (0) of LSMO differs when performing the field sweeps along the field-cooling direction or perpendicular to it reflects the existence of a pinned magnetic domain configuration. Remarkably, the LSMO domain reconfiguration seen in the θ =180° field-sweep data taken in the CIP measurement is reflected over the same field range in the CPP data governed by the vertical transport through the SIO film. It confirms that the magnetic structure of the semiconductor-AFM SIO layer responds to that of the underlying FM LSMO layer, and highlights the exchange-spring magnetic coupling between LSMO and SIO. In Supplementary Fig. 8 and Supplementary Note 8 , we show analogous data to Fig. 4a but obtained after field cooling along θ =180°. The character of the field-sweep magnetoresistance traces measured at θ =180° and θ =90° reverses in Supplementary Fig. 8 as compared with Fig. 4a , which confirms the presence of exchange-coupling at the LSMO/SIO interface and the ‘crystalline’ origin of the AMR. 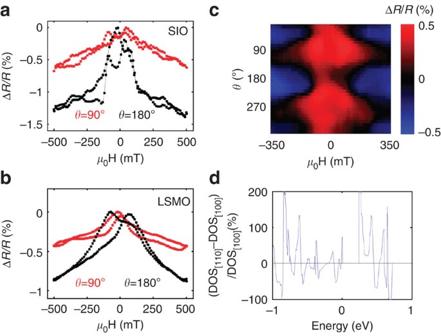Figure 4: Field-dependent magnetoresistance in Sr2IrO4(SIO) and La2/3Sr1/3MnO3(LSMO) and calculated anisotropic density of states. (a) Magnetoresistance of SIO after field-cooling to 4.2 K in applied magnetic field alongθ=90° and subsequently sweeping the magnetic field at the same magnetic field angle and atθ=180°. (b) Same asa, for the lateral LSMO magnetoresistance. (c) Field-sweep magnetoresistance map of SIO for the entire range of field angles. All measurements were performed after the field-cooling alongθ=90°. (d) Relativistic LSDA+U calculations of the in-plane anisotropy of the density of states (DOS), (DOS[110]−DOS[100])/DOS[100]. The calculations demonstrate large overall DOS anisotropies, a significant anisotropy in the band gap and a strong energy dependence of the DOS anisotropy on either side of the band gap of SIO. Figure 4: Field-dependent magnetoresistance in Sr 2 IrO 4 (SIO) and La 2/3 Sr 1/3 MnO 3 (LSMO) and calculated anisotropic density of states. ( a ) Magnetoresistance of SIO after field-cooling to 4.2 K in applied magnetic field along θ =90° and subsequently sweeping the magnetic field at the same magnetic field angle and at θ =180°. ( b ) Same as a , for the lateral LSMO magnetoresistance. ( c ) Field-sweep magnetoresistance map of SIO for the entire range of field angles. All measurements were performed after the field-cooling along θ =90°. ( d ) Relativistic LSDA+U calculations of the in-plane anisotropy of the density of states (DOS), (DOS [110] −DOS [100] )/DOS [100] . The calculations demonstrate large overall DOS anisotropies, a significant anisotropy in the band gap and a strong energy dependence of the DOS anisotropy on either side of the band gap of SIO. Full size image We also point out that, consistently, the magnitude of ΔR ( μ 0 H )/ R (0) in SIO is comparable to the magnitude of the corresponding field rotation AMR signal in SIO (compare Figs 4a and 3a ). Similar experiments to those reported in Fig. 4a,b have been performed over the entire range of angles 0°< θ <360°. The resulting SIO magnetoresistance sweep map, shown in Fig. 4c , has common as well as some distinct features compared with the SIO rotation AMR map in Fig. 3c which are due to the presence of hysteretic effects within the measured field range. We now summarize the experimental evidence that has guided our theoretical analysis presented below. The AMR we observe in our semiconductor-AFM is of the order of 1%. This is a relatively large signal for an Ohmic magnetic device. Moreover, SIO is an easy-plane AFM [15] , whereas the electrical current in the CPP geometry is driven through the SIO film along the out-of-plane c -axis. This implies that for the in-plane field rotations the ‘non-crystalline’ contribution to the AMR, that is, the AMR corresponding to the varying angle between spin-axis and current, does not contribute to our signal in SIO. We are detecting only the ‘crystalline’ AMR because of spin-axis rotation relative to the crystal axes [22] , [24] . Note that this AMR component vanishes in polycrystalline samples as all crystalline contributions average out but can become sizable compared with the non-crystalline AMR in single-crystal magnets with strong spin-orbit coupling [24] . The relatively large crystalline AMR signal we measure in our semiconductor-AFM, comparable to typical non-crystalline AMRs in FMs, confirms high crystal quality of our film and the expected strong spin-orbit coupling effects in SIO. Theory considerations and microscopic calculations Before discussing the microscopic physics of the AFM-AMR in SIO, we recall first the fundamentals of the AMR in FMs. Theoretically, there is a qualitative difference between the microscopic origins of the ohmic non-crystalline and ohmic crystalline AMR components. As the former component depends only on the angle between magnetization and current [22] , the effects of the rotating magnetization on the equilibrium electronic structure do not contribute to the non-crystalline AMR. Instead, in the leading order, the non-crystalline AMR reflects the difference between transport scattering matrix elements of electrons with momentum parallel to the current in the I // m and I ⊥ m configurations [22] , [24] . The difference between scattering matrix elements for an electron with the momentum parallel and perpendicular to the spin axis is due to the relativistic spin-orbit coupling. In the transport geometry corresponding to the pure crystalline AMR, magnetization rotates in the plane perpendicular to the current so that the angle between magnetization and current remains constant and the AMR is determined solely by the varying angle between magnetization and crystal axes. Unlike the non-crystalline AMR, the crystalline AMR originates from the changes in the equilibrium relativistic electronic structure induced by the rotating magnetization. The picture applies not only to the Ohmic regime but also to AMR-like effects, which were more recently discovered in tunnelling [25] , [26] , [27] , [28] , [29] , [30] or single-electron transport devices [31] , [32] , [33] , [34] . In the last case, the anisotropy of the electronic structure with respect to the magnetization angle, or more specifically the anisotropy of the density of states (DOS) and the corresponding position of the chemical potential, provides a direct quantitative description of the measured transport effect [34] . In the case of the tunnelling AMR or the crystalline ohmic AMR, the quantitative relativistic transport theory would require to combine the calculated DOS anisotropy with the tunnelling or scattering matrix elements, respectively. Owing to the anisotropy of the electronic structure with respect to the magnetization angle, the matrix elements may also change when magnetization is rotated. As a proper modelling of these matrix elements for realistic sample parameters is in general a difficult problem, the theories have focused primarily on assessing the qualitative origin of these phenomena based on the DOS calculations as a function of the magnetization angle. We recall that conceptually the AMR phenomena are equally present in AFMs as in FMs [7] . As AMR is an even function of the microscopic magnetic moment vector, it is the direction of the spin-axis rather than the direction of the macroscopic magnetization, which primarily determines the effect. In collinear FMs, the two directions are equivalent. For the staggered spin configuration of compensated AFMs, only the spin-axis can be defined, whereas the macroscopic magnetization is zero. To analyse the electronic structure anisotropy effects with respect to the spin-axis direction in the AFM SIO, we employ the relativistic version of the full-potential linearized augmented-plane wave method [35] . Our in-house full-potential linearized augmented-plane wave code includes the scalar-relativistic and the spin-orbit coupling effects. The spin-orbit coupling is implemented in the self-consistent second-variational procedure [36] . The electron correlation effects are included using the relativistic implementation of rotationally invariant local spin-density approximation with Hubbard parameter U (LSDA+U) method [37] . For Ir atoms, we use the Coulomb parameter U =2.5 eV, and the exchange parameter J =0.26 eV, with the fully localized limit form of the double-counting term. All calculations are done for the experimental lattice constants and internal parameters of SIO with AFM arrangement of the Ir moments [15] , [38] , [39] . Achieving reliable accuracy for the calculated DOS anisotropy in the relativistic LSDA+U method is a significant challenge for bulk SIO and is beyond practical implementation limits for a supercell comprising 102 atoms of the 6 nm SIO slab. In the experiment, we used the thin film SIO to maximize the effect of the LSMO/SIO exchange spring on the SIO AFM spin-axis. However, from the point of view of the basic semiconducting, magnetic and spin-orbit coupling properties of the SIO electronic structure, our thin SIO film is not qualitatively different from bulk SIO, which allows us to assess the qualitative link between the calculated DOS anisotropy and the crystalline AMR based on the bulk SIO calculations. When using the conventional LSDA (with spin-orbit coupling), we obtain a semi-metallic band structure of the SIO with Ir d -like electrons at the M-point and holes at the X-point. In agreement with previous calculations [39] , our results show that LSDA does not provide an appropriate computational model for the electronic structure of SIO and that electron correlation effects and spin-orbit coupling have to be simultaneously included in the modelling. When we employ the relativistic rotationally invariant LSDA+U method, we obtain the semiconductor band structure of SIO. The comparison of LSDA and LSDA+U band structures is shown in Supplementary Fig. 9 and Supplementary Note 9 in and the LSDA+U spin and orbital magnetic moments for the Ir d -states are shown in Supplementary Table 1 and Supplementary Note 9 . We note that other than Ir d -state contributions to the magnetic moment are negligibly small. To analyse the electronic structure anisotropy phenomena, we performed constrained relativistic LSDA+U calculations with the LSDA exchange-correlation field aligned along the [100], [110] and [001] crystal axes. First we inspect the magnetic anisotropy energy, which is evaluated from the difference between total energies for the self-consistent calculations constrained along different axes. The Brillouin zone sampling was varied to ensure the numerical convergence of the magnetic anisotropy. (The use of 405 k -points was found to be sufficient.) The magnetic anisotropy energy differences for the exchange-correlation field aligned along the [001], [100] and [110] are E [001] - E [100] =2.1 meV and E [110] − E [100] =4.2 meV per formula unit. E [100] as the lowest energy state in our calculations is consistent with the experimental in-plane AFM arrangement of SIO. We emphasize that although restricting the LSDA exchange-correlation field along a given crystal axis, there is no explicit constrain on the spin-orbit-coupled LSDA+U occupation matrix. As a result, we also capture the canting effect of the Ir d -state moments from the [100] axis (7.1° for the spin moment and 6.3° for the orbital moment), in agreement with the experimentally observed canted AFM ground state of SIO [15] . In Fig. 4d we plot the calculated in-plane DOS anisotropy, (DOS [110] - DOS [100] )/DOS [100] , which, as explained above, is at the origin of the crystalline AMR phenomena. The anisotropy is remarkably large [7] , as compared, for example, to the previously calculated DOS anisotropies in bimetallic AFMs IrMn and Mn 2 Au,7 and includes a ~10% difference of the size of the band-gap for the [100] and [110] exchange-correlation field directions. As pointed out above, the DOS anisotropy does not quantitatively describe the measured transport anisotropy. Moreover, in our large macroscopic device, inhomogeneities and corresponding averaging effects can be expected to suppress the AMR signal as compared with the calculated DOS anisotropies of an idealized uniform single-crystal SIO. Our theoretical results, nevertheless, clearly demonstrate that sizable crystalline AMR signals can be readily expected in this AFM semiconductor, and that in SIO materials with low impurity concentrations and with microscopic device geometries there is a potential for a large increase of the AMR signal. Finally, we emphasize that the calculated DOS anisotropy strongly varies as a function of energy on either side of the band gap. This directly implies a possibility for a strong electrical gate action on the AMR in the AFM semiconductor. To conclude, semiconductors allow for the control of the density of mobile carriers, and correspondingly the electrical conductivity, by temperature, light, doping or electrostatic gating. Metallic ferromagnets used in spintronic devices allow for a complementary approach in which the electrical current is controlled by manipulating the orientation of electron spins. For more than a decade, the research towards merging the semiconducting and spintronic approaches in one material has focused on utilizing FM semiconductors, which, however, tend to have low magnetic transition temperatures. We have demonstrated that one of the basic spintronics phenomena, namely the AMR, is observed in an AFM semiconductor that opens the possibility to integrate semiconducting and spintronic functionalities by utilizing AFMs. As many AFM semiconductors, unlike FM semiconductors, have high ordering temperatures, our work opens the path towards semiconductor spintronic devices operating at room temperature. In our proof-of-principle device, the utility of a semiconductor-AFM allowed us to simplify the stack, as compared with the metal-AFM TAMR devices, by removing the insulating tunnel barrier. We have employed the strong temperature dependence of transport through the thin film of the SIO semiconductor and demonstrated a transition from a metal-FM to a semiconductor-AFM-governed AMR in the stack. Microscopic calculations presented in our work reveal a strong sensitivity of the electronic structure to the direction of the AFM spin-axis, which explains the observed sizable crystalline AMR in SIO. How to cite this article: Fina, I. et al. Anisotropic magnetoresistance in an antiferromagnetic semiconductor. Nat. Commun. 5:4671 doi: 10.1038/ncomms5671 (2014).